Beryllium-free Li4Sr(BO3)2for deep-ultraviolet nonlinear optical applications Nonlinear optical (NLO) materials are of great importance in laser science and technology, as they can expand the wavelength range provided by common laser sources. Few NLO materials, except KBe 2 BO 3 F 2 (KBBF), can practically generate deep-ultraviolet coherent light by direct second-harmonic generation process, limited by the fundamental requirements on the structure-directing optical properties. However, KBBF suffers a strong layering tendency and high toxicity of the containing beryllium, which hinder the commercial availability of KBBF. Here we report a new beryllium-free borate, Li 4 Sr(BO 3 ) 2 , which preserves the structural merits of KBBF, resulting in the desirable optical properties. Furthermore, Li 4 Sr(BO 3 ) 2 mitigates the layering tendency greatly and enhances the efficiency of second-harmonic generation by more than half that of KBBF. These results suggest that Li 4 Sr(BO 3 ) 2 is an attractive candidate for the next generation of deep-ultraviolet NLO materials. This beryllium-free borate represents a new research direction in the development of deep-ultraviolet NLO materials. Nonlinear optical (NLO) materials, which can halve the wavelength of light (or double the frequency) by second-harmonic generation (SHG) process, are of current interest and great importance in laser science and technology [1] , [2] , [3] . Over the past decades, continuous intensive studies [4] , [5] , [6] , [7] , [8] , [9] , [10] , [11] have resulted in the development of various commercial NLO materials, such as β-BaB 2 O 4 (BBO) [12] , LiB 3 O 5 (ref. 13 ), AgGaS 2 (ref. 14 ) and ZnGeP 2 (ref. 15 ), which are applicable for the generation of coherent light from ultraviolet region to infrared region. However, there is still lack of commercially available NLO materials for the generation of deep-ultraviolet (wavelength below 200 nm) coherent light, limited by the fundamental but conflicting requirements on the structure-directing optical properties [16] : a wide transparency window down to the deep-ultraviolet spectral region, a large SHG response and a sufficient birefringence to achieve phase matchability. Traditionally, the search for deep-ultraviolet NLO materials mainly focused on beryllium borate systems owing to their deep-ultraviolet transparency, thus leading to the discovery of a number of beryllium borates, such as KBe 2 BO 3 F 2 (KBBF) [17] , [18] , SrBe 2 B 2 O 7 (ref. 19 ), Na 2 CsBe 6 B 5 O 15 (ref. 20 ), NaCaBe 2 B 2 O 6 F (ref. 21 ), Na 3 Sr 3 Be 3 B 3 O 9 F 4 (ref. 22 ), NaBeB 3 O 6 and ABe 2 B 3 O 7 (A=K, Rb) [23] . Nevertheless, till now KBBF is the sole material that can practically generate deep-ultraviolet coherent light by direct SHG process. In the structure of KBBF, the NLO-active [BO 3 ] 3− groups in the [Be 2 BO 3 F 2 ] ∞ layers are coplanar and aligned, giving rise to a relatively large SHG response and a sufficient birefringence for the generation of deep-ultraviolet coherent light. Unfortunately, KBBF suffers a strong layering tendency that originates from the weak F − –K + ionic interactions between the adjacent [Be 2 BO 3 F 2 ] ∞ layers, which causes a great difficulty in the growth of thick crystals and thereby severely hinders the NLO performance of KBBF. Moreover, the containing beryllium can cause pneumonia-like symptoms and cancer if inhaled; in this sense, KBBF is not environmentally friendly. Owing to these obstacles, the production of KBBF is still at the stage of laboratory. Therefore, it is urgently demanded to develop the next generation of deep-ultraviolet NLO materials that preserve the merits of KBBF while overcoming the demerits. Here we report a beryllium-free borate, Li 4 Sr(BO 3 ) 2 , whose structure features [SrBO 3 ] ∞ layers bridged by NLO-active [BO 3 ] 3− groups. The [SrBO 3 ] ∞ layers afford [BO 3 ] 3− groups arranged in a manner similar to that in the case of the [Be 2 BO 3 F 2 ] ∞ layers in KBBF, conferring Li 4 Sr(BO 3 ) 2 the optical merits of KBBF. Furthermore, the NLO-active [BO 3 ] 3− groups serving as layer connectors greatly mitigate the layering tendency and, simultaneously, help to enhance the SHG efficiency by more than half as compared with that of KBBF. Crystal growth of Li 4 Sr(BO 3 ) 2 Single crystals of Li 4 Sr(BO 3 ) 2 were grown by the top-seeded solution growth method from a high-temperature melt in the boron-lacking part of the Li 2 O-SrO-B 2 O 3 system (see Fig. 1a and the Methods section). Owing to high corrosion resistance to the melt, Au crucibles were used for the crystal growth instead of Pt crucibles. The melt should be prepared by melting Li 2 CO 3 , SrCO 3 and H 3 BO 3 at a temperature no lower than 1,073 K for 10 h, otherwise Li 2 CO 3 crystals were often obtained. In contrast to KBBF, there is almost no layering tendency observed for Li 4 Sr(BO 3 ) 2 crystal (see Fig. 1b ), and it is relatively easy to obtain thick Li 4 Sr(BO 3 ) 2 crystals. The phase purity was confirmed by powder X-ray diffraction (XRD) and the XRD pattern matches the one calculated from single-crystal XRD analysis very well (see Fig. 1c ). The inductively coupled plasma element analysis of Li 4 Sr(BO 3 ) 2 gave a molar ratio of Li:Sr:B=4.1:1:2.1, which is consistent with the compositions determined by single-crystal XRD analysis. 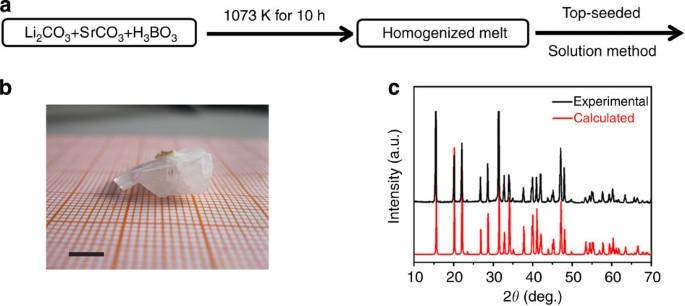Figure 1: Synthesis procedure and XRD patterns for Li4Sr(BO3)2crystal. (a) The synthesis procedure of Li4Sr(BO3)2crystal from high-temperature melt. (b) Photograph of the as-grown Li4Sr(BO3)2crystal. (c) Calculated and experimental XRD patterns for Li4Sr(BO3)2. Scale bar, 5 mm. Figure 1: Synthesis procedure and XRD patterns for Li 4 Sr(BO 3 ) 2 crystal. ( a ) The synthesis procedure of Li 4 Sr(BO 3 ) 2 crystal from high-temperature melt. ( b ) Photograph of the as-grown Li 4 Sr(BO 3 ) 2 crystal. ( c ) Calculated and experimental XRD patterns for Li 4 Sr(BO 3 ) 2 . Scale bar, 5 mm. Full size image Mechanical properties and chemical stability At room temperature, Li 4 Sr(BO 3 ) 2 single crystals with a weight of 0.21 g were exposed in the air for 1 week; they were still transparent and their weight did not change, indicating that Li 4 Sr(BO 3 ) 2 is nonhygroscopic and stable in the air. The measured Vickers hardness of Li 4 Sr(BO 3 ) 2 is 234 Hv, corresponding to Mohs’ hardness at ~3.5. The Li 4 Sr(BO 3 ) 2 crystal has no tendency to cleave and/or crack during cutting and polishing. The good chemical stability and mechanical properties make it easy to process by cutting and polishing. Structural analysis by single-crystal XRD Li 4 Sr(BO 3 ) 2 crystallizes in monoclinic crystal system with an acentric space group of Cc (for detailed crystallographic data, see Supplementary Tables 1–4 ; ORTEP drawing of the asymmetric unit see Supplementary Fig. 1 ). Its structure is composed of two-dimensional [SrBO 3 ] ∞ layers that are further bridged by NLO-active [BO 3 ] 3− groups to construct a three-dimensional framework with Li + cations maintaining the charge balance ( Fig. 2a ). To the best of our knowledge, Li 4 Sr(BO 3 ) 2 is the first NLO material based on two-dimensional [SrBO 3 ] ∞ layers. In the structure of Li 4 Sr(BO 3 ) 2 , there are two crystallographically independent boron atoms, both of which are bound to three oxygen atoms to form planar [BO 3 ] 3− triangles. Each [B1O 3 ] 3− or [B2O 3 ] 3− triangle is distorted with one shortened B–O bond, the B–O distances corresponding to 1.350(12)–1.396(12) Å and 1.365(12)–1.396(11) Å, respectively ( Supplementary Table 3 ). 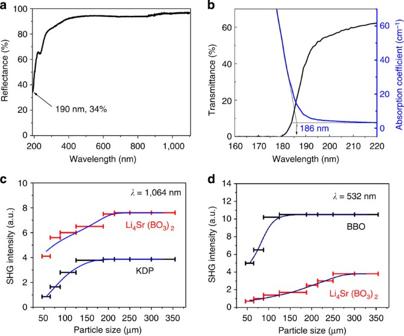Figure 3: Optical properties of Li4Sr(BO3)2. (a) Ultraviolet–visible-near-infrared diffuse reflectance spectrum. (b) Deep-ultraviolet transmission spectrum. (c) SHG intensity as a function of particle size at 1,064 nm. (d) SHG intensity as a function of particle size at 532 nm. KDP and BBO were used as references for the SHG measurements at 1,064 nm and 532 nm, respectively. The black and blue curves inbrepresent the transmittance curve and absorption coefficient curve, respectively. The blue curves incanddare drawn to guide the eyes, and are not fits to the data. Accordingly, the O–B–O angles are in the range of 119. (1)–121.5(8)° and 119.1(8)–120.8(9)°, respectively, showing small deviations from 120° ( Supplementary Table 3 ). The Sr atoms are eight-coordinated to form irregular SrO 8 hexagonal bipyramids ( Fig. 2b ). Each SrO 8 hexagonal bipyramid is linked to three neighbouring [B1O 3 ] 3− triangles by sharing its six equatorial oxygen atoms to further construct a two-dimensional [3, 3] [SrBO 3 ] ∞ layer ( Fig. 2c ) in the ab plane, and simultaneously connects to two [B2O 3 ] 3− triangles by sharing its two apical oxygen atoms to bridge the adjacent [SrBO 3 ] ∞ layers along the c direction. Within a single [SrBO 3 ] ∞ layer, the [3, 3] connection of hexagon SrO 6 and triangular [B1O 3 ] 3− makes all [B1O 3 ] 3− triangles in coplanar and aligned arrangement ( Fig. 2c ). With respect to the layer-connector [B2O 3 ] 3− triangles, they have the opposite orientations to some extent and are approximately parallel to the [SrBO 3 ] ∞ layers with small acute angles. In the structure of Li 4 Sr(BO 3 ) 2 , Li + cations are all four-coordinated ( Supplementary Fig. 2 ) and reside in the cavities of the Li 4 Sr(BO 3 ) 2 configuration to maintain the charge balance ( Fig. 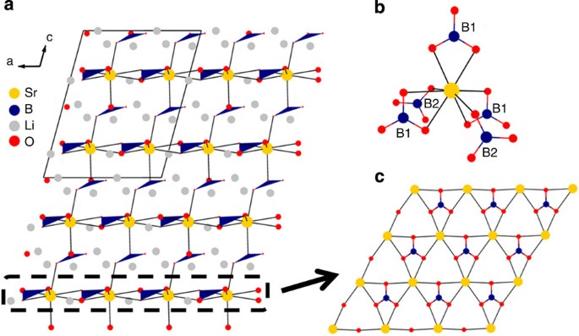2a ). Figure 2: Crystal structural features of Li4Sr(BO3)2. (a) Crystal structure of Li4Sr(BO3)2. (b) [BO3]3−groups coordinated to a SrO8polyhedron. (c) [SrBO3]∞layer. The blue triangles represent [BO3]3−groups. Figure 2: Crystal structural features of Li 4 Sr(BO 3 ) 2 . ( a ) Crystal structure of Li 4 Sr(BO 3 ) 2 . ( b ) [BO 3 ] 3− groups coordinated to a SrO 8 polyhedron. ( c ) [SrBO 3 ] ∞ layer. The blue triangles represent [BO 3 ] 3− groups. Full size image Linear and NLO measurements Ultraviolet–visible–near-infrared diffuse reflectance spectrum ( Fig. 3a ) was collected based on Li 4 Sr(BO 3 ) 2 powders with a PerkinElmer Lamda-900 ultraviolet/visible/near-infrared spectrophotometer in the wavelength range of 190–1,100 nm. The reflectance at 190 nm is ~34%, indicating that the Li 4 Sr(BO 3 ) 2 crystal is transparent to <190 nm. To obtain an accurate value about the ultraviolet absorption edge, deep-ultraviolet transmission spectrum was collected on a Li 4 Sr(BO 3 ) 2 sample ( Supplementary Fig. 3 ) with a McPherson VUVas2000 spectrophotometer in the wavelength range of 120–220 nm. As shown in Fig. 3b , the deep-ultraviolet absorption edge is located at 186 nm, indicating that the Li 4 Sr(BO 3 ) 2 crystal is suitable for deep-ultraviolet applications. As Li 4 Sr(BO 3 ) 2 crystallizes in an acentric space group, it is expected to possess NLO properties. We carried out visible and ultraviolet SHG measurements by the Kurtz–Perry method [24] with incident lasers at λ =1,064 and λ=532 nm, respectively. Meanwhile, the well-known NLO materials KH 2 PO 4 (KDP) and BBO were used as references, respectively. The curves of SHG signal as a function of particle size are also shown in Fig. 3 . The SHG intensities increase with increasing particle sizes before they attain the maximization independent of the particle sizes in both Fig. 3c,d , indicating that Li 4 Sr(BO 3 ) 2 is phase matchable in both visible and ultraviolet region. Despite a large number of borate NLO materials being ultraviolet transparent, only a few of them are phase matchable in the visible region, and fewer are phase matchable in the ultraviolet region. Moreover, Li 4 Sr(BO 3 ) 2 exhibits a large SHG efficiency ~2.0 times that of KDP in the same particle size of 214–250 μm with the incident laser at 1,064 nm (see Fig. 3c ). With the incident laser at 532 nm, the SHG intensity of Li 4 Sr(BO 3 ) 2 is about one third that of BBO in the same particle size of 214–250 μm (see Fig. 3d ). Considering d 36 (KDP)=0.38 pm V −1 and d 11 (BBO)=2.2 pm V −1 (ref. 25 ), the relative magnitude of SHG efficiency in the visible region and that in the ultraviolet region are consistent with each other, and the derived d eff coefficient for Li 4 Sr(BO 3 ) 2 is ~0.76 pm V −1 , which is ~1.6 times that of KBBF ( d 11 =0.47 pm V −1 ) [26] . Taking the weak layering tendency and enhanced SHG efficiency into account, in comparison with KBBF, Li 4 Sr(BO 3 ) 2 probably exhibits much higher NLO performance in practical applications. Figure 3: Optical properties of Li 4 Sr(BO 3 ) 2 . ( a ) Ultraviolet–visible-near-infrared diffuse reflectance spectrum. ( b ) Deep-ultraviolet transmission spectrum. ( c ) SHG intensity as a function of particle size at 1,064 nm. ( d ) SHG intensity as a function of particle size at 532 nm. KDP and BBO were used as references for the SHG measurements at 1,064 nm and 532 nm, respectively. The black and blue curves in b represent the transmittance curve and absorption coefficient curve, respectively. The blue curves in c and d are drawn to guide the eyes, and are not fits to the data. Full size image First-principles calculations To elucidate the mechanism of optical properties in Li 4 Sr(BO 3 ) 2 , the first-principles calculations were performed by the plane-wave pseudopotential method implemented in the CASTEP package based on the density functional theory [27] , [28] , [29] . 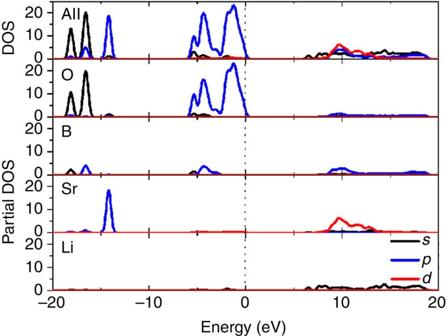Figure 4: DOS and partial DOS plots for Li4Sr(BO3)2. DOS plots of Li4Sr(BO3)2, and partial DOS plots of the respective species in Li4Sr(BO3)2. Figure 4 displays the density of states (DOS) and partial DOS of the respective species in Li 4 Sr(BO 3 ) 2 . Evidently, in these states the contribution from the orbitals of the Li + and Sr 2+ cations is negligibly small, despite that the orbitals of the larger Sr 2+ cations become slightly significant at the bottom of the conduction band. The valence band top (−6 to 0 eV) and conduction band bottom (6–12 eV) are mainly composed of the O 2 p and B 2 p orbitals, respectively, indicating that the optical transition between these states (in the [BO 3 ] 3− groups) does dominate the principal optical properties, for example, refractive indices and SHG coefficients, of Li 4 Sr(BO 3 ) 2 . Based on the electronic band structures ( Supplementary Fig. 4 ), the dispersions of the linear refractive indices ( Supplementary Fig. 5 ) for Li 4 Sr(BO 3 ) 2 were calculated. The derived birefringence is Δ n =0.056 (at an incident wavelength of 532 nm), which is close to that of KBBF (Δ n =0.070) [26] . Clearly, such a large birefringence is sufficient for the phase matchability in the visible and ultraviolet region. The phase-matching conditions have been deduced from the calculated refractive indices, as shown in Supplementary Table 5 , which confirms that Li 4 Sr(BO 3 ) 2 is phase matchable for SHG of 1,064 and 532 nm lasers. The SHG coefficient d ij was calculated by the formula developed by Lin et al . [30] , [31] As Li 4 Sr(BO 3 ) 2 belongs to the monoclinic crystal system with a space group of Cc , it has six non-zero independent SHG coefficients. The largest two SHG coefficients for Li 4 Sr(BO 3 ) 2 are d 11 =−0.71 pm V −1 and d 12 =0.64 pm V −1 , respectively (all SHG coefficients see Supplementary Table 6 ), which are in good agreement with the derived d eff coefficient (~0.76 pm V −1 ) by powder SHG measurements. Figure 4: DOS and partial DOS plots for Li 4 Sr(BO 3 ) 2 . DOS plots of Li 4 Sr(BO 3 ) 2 , and partial DOS plots of the respective species in Li 4 Sr(BO 3 ) 2 . Full size image Atom-cutting analysis To further analyse the contribution of an ion (or an anionic group) to the birefringence and SHG response, a real-space atom-cutting technique [32] , [33] was adopted. Herein, the largest two SHG coefficients are selected for the sake of comparison (the full analysis for birefringence and SHG coefficients see Supplementary Tables 6 and 7 , respectively). As shown in Table 1 , the anionic B–O groups ([B1O 3 ] 3− and [B2O 3 ] 3− ) make the dominant contributions to both SHG coefficients and birefringence, while the contributions of the alkaline and alkaline earth cations (Li + and Sr 2+ ) are negligibly small. The results are well consistent with the partial DOS analysis. Moreover, the layer-connector [B2O 3 ] 3− groups contribute smaller to the birefringence and SHG coefficients as compared with the [B1O 3 ] 3− groups in the [SrBO 3 ] ∞ layers. Table 1 Atom-cutting analysis and calculated birefringence and SHG coefficients at 532 nm. Full size table The optical properties can also be elucidated from the structural features in Li 4 Sr(BO 3 ) 2 . According to the anionic group theory [32] , for alkaline or alkaline-earth borate B–O groups are the dominating active units, which determine the birefringence and SHG coefficient. In the structure of Li 4 Sr(BO 3 ) 2 , the compositional [B1O 3 ] 3− groups of [SrBO 3 ] ∞ layers and the layer-connector [B2O 3 ] 3− groups are approximately in the same plane normal to the c axis with small dihedral angles of 22.88(17)° and 20.73(17)°, respectively. Thus, it is reasonable that both [B1O 3 ] 3− and [B2O 3 ] 3− groups contribute a lot to the anisotropic optical response, that is, birefringence. The resultant birefringence (Δ n =0.056) is also reasonable, considering that the perfect coplanar [BO 3 ] 3− arrangement in KBBF gives rise to a larger birefringence of about Δ n =0.070. In terms of SHG properties, the [B1O 3 ] 3− groups in the [SrBO 3 ] ∞ layers are arranged in a constructively added manner to give the major contribution to the SHG coefficients. In addition, despite for the layer-connector [B2O 3 ] 3− groups the microscopic second-order susceptibilities have a partial cancellation arising from the somewhat opposite arrangement, they are not completely offset. As a result, the layer connectors also make considerable contributions to the SHG coefficients. In other words, they help to further enhance the SHG efficiency by more than half as compared with that of KBBF. It is well known that the overall nonlinearity of a crystal is the geometrical superposition of the microscopic second-order susceptibility of the NLO-active anionic groups [32] . Taking the layer-connector [BO 3 ] 3− groups into account, the overall number density of [BO 3 ] 3− groups is 0.0148 per unit volume for Li 4 Sr(BO 3 ) 2 , which is ~1.57 times that of KBBF (0.00946 per unit volume). It is also well known that distorted anionic groups (for example, [BO 4 ] 5− tetrahedra in SrB 4 O 7 (ref. 1 ), [TiO 6 ] 8− octahedra in KTiOPO 4 (ref. 33 ) and [NbO 6 ] 7− octahedra in LiNbO 3 (ref. 34 )) possess larger microscopic second-order susceptibilities than that of regular ones. In Li 4 Sr(BO 3 ) 2 , every [BO 3 ] 3− group is somewhat distorted with one shortened B–O bond; hence, they are presumable to have larger microscopic second-order susceptibilities in comparison with the regular ones in KBBF. Consequently, the distortion of [BO 3 ] 3− groups well compensate the partial cancellation of microscopic second-order susceptibilities of the layer connectors, resulting in an overall SHG coefficient ~1.6 times as large as that of KBBF. Structurally, the [SrBO 3 ] ∞ layers are closely related to the [Be 2 BO 3 F 2 ] ∞ layers (in the structure of KBBF) where the [3, 3] connection of tetrahedral BeO 3 F and triangular [BO 3 ] 3− makes [BO 3 ] 3− triangles arrange in a coplanar and aligned manner [26] , indicating that the Li 4 Sr(BO 3 ) 2 crystal has a high potential to inherit the optical merits of KBBF (including a relatively large SHG response and a sufficient birefringence). Meanwhile, compared with KBBF where the layered structural units are weakly connected by the F − –K + ionic bonds resulting in a strong layering tendency, the connection between [SrBO 3 ] ∞ layers in Li 4 Sr(BO 3 ) 2 are largely reinforced by the [B2O 3 ] 3− groups serving as bridges. This point can be elucidated by calculating the electrostatic force of interactions between the layered structural units. In the structure of Li 4 Sr(BO 3 ) 2 , the layer-connector [B2O 3 ] 3− groups act as rigid building units owing to their covalent B–O bonds; thus, the interactions between [SrBO 3 ] ∞ layers are dominated by the Sr–O bonds that are basically ionic. According to Coulomb’s law [35] , the magnitude of the electrostatics force of interaction can be calculated using the equation (1): where k e is the electrostatic constant, q 1 and q 2 are the magnitude of the two point charges, respectively, and r is the separation distance between point charges. The calculated value for | F ( Sr 2+ - O 2- ) | is ~4.7 times as large as that of | F ( K + - F - ) | , revealing a largely reinforced layer connection for Li 4 Sr(BO 3 ) 2 in comparison with that in KBBF. In our preliminary attempts of crystal growth, almost no layering tendency was observed, which experimentally confirms the aforementioned analysis based on microscopic crystal structure. In summary, we have synthesized a new beryllium-free borate, Li 4 Sr(BO 3 ) 2 , which consists of [SrBO 3 ] ∞ layers that are further bridged by NLO-active [BO 3 ] 3− groups to form a three-dimensional framework with Li + cations maintaining the charge balance. The [SrBO 3 ] ∞ layers inherit the structural merits of KBBF, and the [BO 3 ] 3− groups serving as layer connectors help to enhance the SHG efficiency by more than half as compared with that of KBBF. As a result, Li 4 Sr(BO 3 ) 2 exhibits a deep-ultraviolet absorption edge at 186 nm and is phase matchable not only in the visible region but also in the ultraviolet region, with a powder SHG efficiency of ~2.0 × KDP (or ~1.6 × KBBF) at 1,064 nm. Meanwhile, Li 4 Sr(BO 3 ) 2 mitigates the layering tendency to a great extent by reinforcing the electrostatics interactions between the layered structural units to ~4.7 times that of KBBF in magnitude. Combining the weak layering tendency with an enhanced SHG efficiency, Li 4 Sr(BO 3 ) 2 may exhibit much higher NLO performance than KBBF in practical applications. All the compositional elements are nontoxic, indicating that Li 4 Sr(BO 3 ) 2 is environmentally friendly. Therefore, Li 4 Sr(BO 3 ) 2 is an attractive candidate for the next generation of deep-ultraviolet NLO materials. This beryllium-free borate represents a new research direction in the development of deep-ultraviolet NLO materials, as the traditional materials generally contain beryllium. Synthesis of Li 4 Sr(BO 3 ) 2 Crystals Single crystals of Li 4 Sr(BO 3 ) 2 were grown by the top-seeded solution growth method from a high-temperature Li 2 O/SrO/B 2 O 3 melt. This melt was prepared by melting a mixture of 177.4 g (2.40 mol) Li 2 CO 3 , 59.0 g (0.40 mol) SrCO 3 and 74.2 g (1.20 mol) H 3 BO 3 (at a molar ratio of Li 2 O:SrO:B 2 O 3 =12:2:3). Li 2 CO 3 (98.0%), SrCO 3 (99.0%) and, H 3 BO 3 (99.5%) were used as received. The mixture was placed into a Φ 60 × 60 mm Au crucible, rapidly heated to 1,073 K in a temperature-programmable electric furnace and then held for no <10 h to ensure that the carbonates were decomposed and the melt was homogenized. In the first run of growth, a Au wire was dipped into the melt to serve as a nucleation centre. The temperature was decreased at a rate of 5 K h −1 until Li 4 Sr(BO 3 ) 2 crystals nucleared on the Au wire. In the following run of growth, the saturation temperature was determined by a tentative seed crystal method. A seed crystal obtained in the first run was attached to a Au rod and then slowly dipped into the melt surface at 10 K above the saturation temperature. The temperature was held for 60 min to dissolve the rough surfaces of the seed crystal and then was decreased to the saturation temperature within 10 min before the melt was allowed to cool at a rate of 0.5–2.0 K per day. The crystal was rotated at a rate of 25 r.p.m. during the growth process. When the growth finished, the crystal was drawn out of the melt and then cooled down to room temperature at a rate of 20 K h −1 . The as-grown Li 4 Sr(BO 3 ) 2 crystal with dimensions of 17 × 15 × 4 mm 3 is shown in Fig. 1b . Powder XRD analysis confirmed the phase purity ( Fig. 1c ) and the elemental analysis confirmed the molar ratio of Li/Sr/B as 4.1/1/2.1. Physical measurements Powder XRD analysis was carried out at room temperature on a Rigaku MiniFlex II diffractometer equipped with Cu K α radiation. The Vickers hardness measurement was carried out with the as-grown crystal and on a HX-1000TM Type Vickers hardness tester. The measurement was performed at room temperature and the maximum load applied for Li 4 Sr(BO 3 ) 2 crystal was 50 g with an indentation time of 10 s. Elemental analysis was performed by using a Jobin Yvon Ultima2 inductively coupled plasma optical emission spectrometer with Sepex Certiprep standards. The single-crystal XRD data were collected by using graphite-monochromatized Mo K α radiation ( λ =0.71073 Å) at 293 (2) K on a Rigaku Saturn70 diffractometer equipped with a Saturn CCD detector. The collection of the intensity data, cell refinement and data reduction were carried out with the programme Crystalclear [36] . The structure was solved by the direct method with the programme SHELXS and refined with the least-squares programme SHELXL of the SHELXTL.PC suite of programmes [37] . Final refinement includes anisotropic displacement parameters. The structure was verified using the ADDSYM algorithm from the programme PLATON [38] and no higher symmetries were found. The ultraviolet –visible–near-infrared diffuse reflection data in the wavelength range of 190–1,100 nm were recorded at room temperature using a powder sample with BaSO 4 as a standard (100% reflectance) on a PerkinElmer Lamda-900 ultraviolet /visible/near-infrared spectrophotometer. The deep-ultraviolet transmission spectrum was measured at room temperature using a spectrophotometer (VUVas2000, McPherson) in the wavelength range of 120–220 nm. A transparent Li 4 Sr(BO 3 ) 2 sample with a thickness of ~1 mm ( Supplementary Fig. 3 ) was cut from the as-grown crystal ( Fig. 1b ) and polished to optical grade for the deep-ultraviolet measurement. The absorption coefficient α is determined from the formula α =[2ln(1− R )−ln T ]/ l (ref. 39 ), where T is the transmissivity, R is the reflectivity and l is the sample thickness. Here the T- values can be directly obtained from experiments, but the R -values is difficult to obtain, as R =( n −1) 2 /( n +1) 2 (ref. 39 ) and the measured refractive indices are not available. To overcome this problem, we adopted the refractive indices obtained by the first-principles calculations in the reflectivity calculations. Our previous studies have clearly demonstrated that the absolute error between the experimental and first-principles refractive indices is typically <0.1 for ultraviolet and deep-ultraviolet NLO borates [40] . This small error would result in the uncertainty of the reflectivity and absorption coefficients <2% and 0.1 cm −1 , respectively, in the Li 4 Sr(BO 3 ) 2 crystal. Powder SHG measurements were carried out by the Kurtz–Perry method [24] . The measurements were performed with a laser at 1,064 nm and a frequency doubling at 532 nm, for visible and ultraviolet SHG, respectively. Polycrystalline Li 4 Sr(BO 3 ) 2 samples were ground and sieved into the following particle size ranges: 46–65, 65–88, 88–125, 125–188, 188–214, 214–250, 250–300 and 300–355 μm. KDP and BBO were also ground and sieved into the same particle size ranges and used as references for visible and ultraviolet SHG tests, respectively. Computational methods The first-principles calculations for the electronic structures in Li 4 Sr(BO 3 ) 2 were performed by the plane-wave pseudopotential method implemented in the CASTEP package based on the density functional theory [27] , [28] , [29] . The ion–electron interactions were modelled by the optimized normal-conserving pseudopotentials [41] and the local density approximation [27] was chosen for all the calculations. The kinetic energy cutoff of 900 eV and the Monkhorst–Pack k -point meshes [42] with a density of (4 × 4 × 2) points in the Brillouin zone were adopted. Our tests reveal that the above computational set-ups are sufficiently accurate for present purposes. Based on the obtained electronic structures, the linear and NLO properties for Li 4 Sr(BO 3 ) 2 were calculated. The linear optical refractive indices and birefringence can be obtained from the electronic transition between the occupied and unoccupied states caused by the interaction with photons [43] . The SHG coefficient d ij was calculated by the formula developed by Lin et al. [30] , [31] It is well acknowledged that the local density approximation calculations always underestimate the energy band gap of crystals. Thus, a scissors operator [44] was introduced to shift up all the conduction bands to agree with the measured band gap. To analyse the contribution of an ion (or an anionic group) to the n th order susceptibility χ (n) , a real-space atom-cutting technique was adopted [30] , [31] . Within this method the contribution of ion A to the n th-order susceptibility (denoted as χ ( n ) ( A )) can be obtained by cutting all ions except A from the original wave functions χ (n ) ( A )= χ ( n ) (all ions except A are cut). How to cite this article: Zhao, S. et al. Beryllium-free Li 4 Sr(BO 3 ) 2 for deep-ultraviolet nonlinear optical applications. Nat. Commun. 5:4019 doi: 10.1038/ncomms5019 (2014).